Atomic-scale engineering of magnetic anisotropy of nanostructures through interfaces and interlines The central goals of nanoscale magnetic materials science are the self-assembly of the smallest structure exhibiting ferromagnetic hysteresis at room temperature, and the assembly of these structures into the highest density patterns. The focus has been on chemically ordered alloys combining magnetic 3 d elements with polarizable 5 d elements having high spin–orbit coupling and thus yielding the desired large magneto-crystalline anisotropy. The chemical synthesis of nanoparticles of these alloys yields disordered phases requiring annealing to transform them to the high-anisotropy L1 0 structure. Despite considerable efforts, so far only part of the nanoparticles can be transformed without coalescence. Here we present an alternative approach to homogeneous alloys, namely the creation of nanostructures with atomically sharp bimetallic interfaces and interlines. They exhibit unexpectedly high magnetization reversal energy with values and directions of the easy magnetization axes strongly depending on chemistry and texture. We find significant deviations from the expected behaviour for commonly used element combinations. Ab-initio calculations reproduce these results and unravel their origin. As feature sizes get smaller, more and more atoms are located at interfaces. Mostly, these interfaces are two-dimensional (2D); however, for sub-10 nm structures, a significant fraction of the atoms are located at one-dimensional (1D) interlines. There is a wealth of fascinating material properties emerging from inversion symmetry breaking and hybridization of electronic states at interfaces. Prominent examples are interface-induced superconductivity [1] , [2] , ferroelectricity [3] , room temperature multiferroicity [4] , strongly correlated electron gases at the interface between two oxides [5] , topological insulators [6] , the Rashba effect [7] , [8] , [9] , the spin–orbit torque effect [10] , [11] , the exchange bias effect [12] , [13] , [14] , and magnetic interface anisotropies [15] , [16] , [17] , [18] , [19] , [20] , [21] . We focus on the latter and investigate model systems grown with atomic level control, enabling a fundamental understanding of interface and interline magnetic anisotropies and reveal their potential in the atomic-scale control and design of future magnetic materials. Although former works revealed the role of the atomic coordination number, that is, the magnetic anisotropy of atoms facing vacuum [22] , [23] , we focus here on the role of coordination chemistry and texture, enabling the optimal employment of all constituent atoms and the construction of embedded magnetic nanostructures. We studied mono- and bilayer islands <1,200 atoms in size and grown on a Pt(111) surface. Atomically sharp 1D interlines have been investigated in core–shell structures with Pt- and Co-cores surrounded by Fe-, Co-, Pt- or Pd shells. Co/Fe interlines yield an increase of the magnetic hardness by 70% as compared with pure Co islands, whereas Co/Pt and Co/Pd interlines reduce it by 60%. A random Fe 0.5 Co 0.5 alloy increases the anisotropy by less than a single Co/Fe interline. The effect of 2D interfaces on the magnetic hardness has been investigated by capping the islands. Capping pure Co islands with a single Pd layer more than doubles the magnetic hardness. The interline effect is found to be preserved after capping. Thus, interline and interface anisotropies can be added up to optimally tune the island blocking temperature. This is illustrated by an example where the magnetic hardness is increased by 160%. Enhancing the island blocking temperature by 1D interlines The parameter most relevant for applications in magnetic information storage is the magnetic anisotropy energy and the resulting thermal stability of the magnetization expressed by the blocking temperature T b . It is defined by the temperature where the imaginary part of the zero-field susceptibility χ″( T ) takes on its maximum and depends on the time scale of the measurement. Below T b the magnetization retains its orientation enabling non-volatile information storage, whereas above it reverses by thermal excitation giving rise to superparamagnetism. We first demonstrate how sensitive T b depends on the chemistry of atomically sharp interlines. 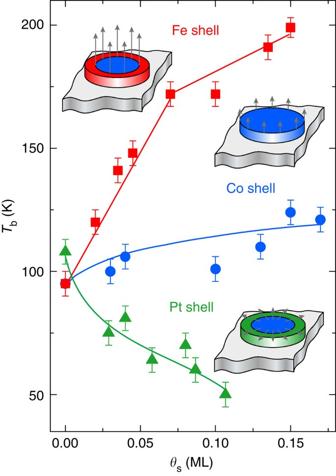Figure 1: Chemical difference of interline anisotropy. Blocking temperatureTbof Co-core islands as a function of the shell coverage Θsand element, Fe (red), Co (blue) and Pt (green). Lines are guides to the eye and error bars reflect the uncertainty of the χ″(T) peak position. For simplicity, we drew the islands circular, the real ones are more irregular, as shown inSupplementary Fig. S1. The arrows represent the direction and magnitude of the magnetic anisotropy emerging from the respective interlines. Growth of Co-cores: coverage Θc=0.12 ML for Fe shells and 0.18 ML for Pt shells, 1 ML is defined as one atom per Pt(111) substrate atom, deposition fluxFCo=0.18±0.01 ML min−1, deposition temperatureTdep=150 K, annealing temperatureTann=250 K; growth of shells:Tdep=250 K,FFe=0.12±0.01 ML min−1,FPt=0.009±0.001 ML min−1. Figure 1 shows magneto-optical Kerr effect (MOKE) measurements for one atomic monolayer (ML) high Co islands adsorbed on a Pt(111) surface. The islands have irregular shape ( Supplementary Fig. S1 ) and out-of-plane easy magnetization axis. They have been surrounded by shells creating a lateral interline between the Co core and the respective shell element. Figure 1: Chemical difference of interline anisotropy. Blocking temperature T b of Co-core islands as a function of the shell coverage Θ s and element, Fe (red), Co (blue) and Pt (green). Lines are guides to the eye and error bars reflect the uncertainty of the χ″( T ) peak position. For simplicity, we drew the islands circular, the real ones are more irregular, as shown in Supplementary Fig. S1 . The arrows represent the direction and magnitude of the magnetic anisotropy emerging from the respective interlines. Growth of Co-cores: coverage Θ c =0.12 ML for Fe shells and 0.18 ML for Pt shells, 1 ML is defined as one atom per Pt(111) substrate atom, deposition flux F Co =0.18±0.01 ML min −1 , deposition temperature T dep =150 K, annealing temperature T ann =250 K; growth of shells: T dep =250 K, F Fe =0.12±0.01 ML min −1 , F Pt =0.009±0.001 ML min −1 . Full size image It is seen that minute amounts of Fe steeply increase T b , whereas a Pt shell strongly reduces it. The increase for Fe is undoubtedly caused by the Co/Fe interline as the curve takes on a smaller slope from a shell coverage of Θ s, Fe =0.07 ML on, where the Fe rim is on average two atoms wide. At that point T b has increased by 55% compared with pure Co islands of the same size shown for comparison, at Θ s, Fe =0.15 ML the increase is 70%. The strong reduction caused by the Co/Pt interline is unexpected in view of the large magneto-crystalline out-of-plane anisotropy emerging from a close-packed interface between the two elements [24] . Therefore, interlines and interfaces between the same elements cause quite different anisotropy. The blocking temperatures are linked to activation energies E for thermal magnetization reversal by with f the sweep frequency of the field and ν 0 the pre-exponential factor that we set to a typical value of ν 0 =2 × 10 10 Hz [25] , [26] . As pure Co and Fe have very similar anisotropy on Pt(111) (see Fig. 4 below and Moulas et al . [27] ), we attribute the Fe shell-induced T b increase solely to the Co/Fe interline and find E il, Co−Fe =0.61±0.10 meV per atomic length of the interline, which we will call per atom in what follows. For the Co/Pt interline we determine E il, Co−Pt =−0.44±0.10 meV/atom under the assumption of homogeneous decoration of the Co-cores for Θ s =0.07 ML. The relationship of these energies with the magnetic anisotropy K depends on the magnetization reversal mechanism. For coherent rotation of all magnetic moments E = K (ref. 25 ), while for domain wall nucleation and propagation this relationship depends on the island shape, for example, for elongated nanostructures it is (ref. 28 ). K is the sum of the magneto-crystalline anisotropy of the island K mc , of the one induced in the substrate K mc, Pt , and of the shape anisotropy K s . We performed fully relativistic ab-initio calculations of all three quantities and find that the latter two contributions are comparatively small and of opposite sign, almost compensating each other. We therefore concentrate our discussion of the origin of the strong, and for Pt shells unexpected sign of the interline-induced magnetic hardness on the theoretical K mc results. Strain and electronic structure may both contribute to K mc . Concerning strain, our STM results show the absence of partial dislocations revealing that the majority of the Fe and Co atoms are pseudomorphic to the substrate despite the large lattice misfit of −10.3 % for Fe and −9.4 % for Co. For Fe this is expected as it grows pseudomorphic on Pt(111) up to completion of the first monolayer [29] . For Co, the appearance of dislocations depends on size [27] , [30] . The present islands with irregular shape stay pseudomorphic up to 1,000 atoms. Following these observations, the lateral atomic positions were chosen to be pseudomorphic in the calculations. We are well aware that this is a simplification as the stress is expected to be partly relieved at the island edges [31] . The interlayer distance has been fixed to the Pt(111) value as this enables to approach the experimental island size with an affordable computational effort. We show for smaller islands in Supplementary Fig. S2 that vertical relaxation changes the absolute numbers but not the general trend that we aim to understand. 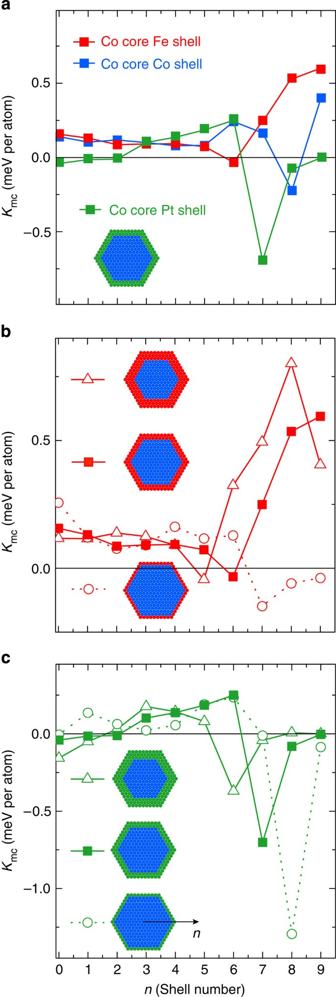Figure 2: Calculated shell-resolved magneto-crystalline anisotropy energy for hexagonal islands containing 271 atoms. (a) AtomicKmcvalues averaged over concentric hexagonal atomic shells with labelnincreasing in going out from the island centre for Co core Fe- (red), Co- (blue) and Pt shell (green) islands for a shell width of two atoms. (b,c) Effect of shell width onKmcfor one atom- (open circles), two atom- (full squares) and three atom-(open triangles) wide Fe (b) and Pt (c) shells, respectively (island diameter 4.71 nm). Figure 2 presents atomic shell-resolved K mc values for hexagonal core–shell islands with 271 atoms on Pt(111). Figure 2a focuses on the effect of the shell chemistry, whereas Figs 2b address the effect of the shell width for Fe and Pt, respectively. Figure 2a shows that K mc has an almost constant and small value from the centre up to two atoms before the interline, from where on a dramatic chemical difference becomes evident. For Fe, K mc reaches 0.6 meV/atom for both atomic rows of the shell. For pure Co, the maximum anisotropy is obtained for edge atoms only, in agreement with Rusponi et al . [23] . By going towards the centre by one atom, K mc jumps to negative values, then back to large positive values for the next two rows until it enters the constant regime. For Pt, both shell atoms have almost no anisotropy and the anisotropy of Co atoms interfacing Pt evaluates to −0.7 meV/atom. All values are without the contribution of the Pt substrate, including it produces a constant upward shift by about 0.17 meV/atom for all curves. Figure 2: Calculated shell-resolved magneto-crystalline anisotropy energy for hexagonal islands containing 271 atoms. ( a ) Atomic K mc values averaged over concentric hexagonal atomic shells with label n increasing in going out from the island centre for Co core Fe- (red), Co- (blue) and Pt shell (green) islands for a shell width of two atoms. ( b , c ) Effect of shell width on K mc for one atom- (open circles), two atom- (full squares) and three atom-(open triangles) wide Fe ( b ) and Pt ( c ) shells, respectively (island diameter 4.71 nm). Full size image For Fe a shell width of two atoms is required for the appearance of the interline anisotropy, as seen in Fig. 2b , whereas for Pt the interline anisotropy is already present for a one atom-wide shell ( Fig. 2c ). A monatomic Fe shell reduces the anisotropy of the two outermost Co rows to negative values, also the Fe shell atoms themselves have negative anisotropy. In contrast, a diatomic Fe shell gives rise to large positive anisotropy for both shell atoms and the Co atom at the interface. The K mc profile of an island with triatomic Fe-shell resembles the diatomic one, it is shifted by one atom towards the island centre and the outermost Fe atom has a reduced anisotropy. In contrast, Pt decoration induces a negative anisotropy in the interfacing Co atoms independent of shell width; however, with the strongest effect for a single-atom shell and weaker effect for thicker shells. Summing K mc over all constituent atoms, and including the contribution of the Pt substrate, we get a total K mc =108 meV for a two atom-wide Fe-shell Co-core island, which is 48% larger than the value of 73 meV obtained for a pure Co island of the same size and shape. This increase is almost identical with the experimental one in T b . Finally, we find K mc =17 meV for a di-, and −18 meV for a monatomic Pt-shell Co-core island. To establish a close comparison with experiment, we transferred the shell-resolved ab-initio K mc values to the experimental island sizes and shapes. For this, we simulated the atomic morphology of the islands by means of kinetic Monte–Carlo [32] with parameters reproducing the experimental island densities and shapes for all three elements ( Supplementary Fig. S1 , and Supplementary Methods ). The simulations yield the abundance of atoms as a function of their coordination chemistry. Adding up the calculated magnetic anisotropies over all constituent atoms produces the theoretical anisotropies per island shown in Fig. 3 as function of shell thickness. For a Co-core Fe-shell island, K mc (Θ s ) shows an initial small dip followed by a steep increase up to a shell coverage of 0.07 ML, where the slope significantly decreases. For a Co-core Pt-shell island the calculated anisotropy energy strongly decreases with increasing Pt coverage, and the pure Co islands show a linear curve located between the ones for Fe and Pt shells. 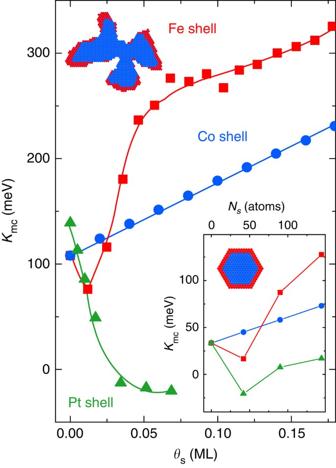Figure 3: Calculated magneto-crystalline anisotropy energy for experimental island sizes and shapes. We have added the shell-resolved atomicKmcvalues fromFig. 2, according to the abundance of correspondingly coordinated atoms in kinetic Monte–Carlo (KMC)-simulated experimental core–shell islands. Inset: total anisotropy energy, including the anisotropy of the magnetic moments induced in the Pt substrate, calculated for hexagonal core–shell islands as a function of shell width for Fe-, Co- and Pt shells; the Co core consists of 127 atoms. Figure 3: Calculated magneto-crystalline anisotropy energy for experimental island sizes and shapes. We have added the shell-resolved atomic K mc values from Fig. 2 , according to the abundance of correspondingly coordinated atoms in kinetic Monte–Carlo (KMC)-simulated experimental core–shell islands. Inset: total anisotropy energy, including the anisotropy of the magnetic moments induced in the Pt substrate, calculated for hexagonal core–shell islands as a function of shell width for Fe-, Co- and Pt shells; the Co core consists of 127 atoms. Full size image The calculated K mc —and the measured T b —curves of Fig. 1 compare very well for each core–shell combination, showing that the shell chemistry effect is astonishingly well reproduced. We chose to present K mc values and not calculated T b values as this would require assumptions on the reversal mechanism. To get nevertheless a feeling for absolute numbers, we calculate T b for one example, namely a Co core 0.07 ML Fe-shell island, and under the assumption of coherent magnetization reversal. The resulting T b =148 K is surprisingly close to the experimental value of 170 K. As seen from Supplementary Fig. S2 , vertical relaxations enhance K mc of the Co/Fe interline and thus approach experiment and theory even further. There are a few differences between experiment and theory on which we would like to comment. The small local minimum of the calculated Fe-shell curve at 0.015 ML is absent in experiment. We attribute this discrepancy to the fact that the calculations have been performed for straight steps, while the experimental islands have rough steps implying atoms with a large variation of coordination number with different K mc values. The linear increase of K mc for the pure Co islands is removed by vertical relaxation, see Supplementary Fig. S2 . The negative K mc values found for large Pt shells are at odd with experiment. This difference is partly removed by taking substrate-induced and shape anisotropy into account ( K mc, Pt =0.17±0.01 and K s, Co =−0.12±0.01 meV/atom in the island centre). These differences in details cannot mask the overall success of theory reproducing the interline chemistry and the fact that two atom-wide shells are needed for the Fe/Co interline magnetic hardness to fully develop. Homogeneous alloy versus 1D interlines We now compare the anisotropy of sharp Co/Fe interlines with one of the nanostructures made of alloys of the two elements. This way, we determine whether homogeneous alloys or onion-like alternations of elements are giving higher magnetic hardness. A meaningful comparison requires alloy composition-independent atomic-scale morphology, that is, the Fe x Co 1− x island areas, and due to the strong effect of atomic coordination [22] , [23] also their perimeter lengths and shapes, have to be identical for 0≤ x ≤1. Co-deposition of both elements results in strongly composition-dependent island densities and shapes due to the different diffusion barriers of both elements. Therefore, we nucleated the Fe x Co 1− x alloy at Pt cores. The insert in Fig. 4a shows that the alloy shell areas A s and their outer perimeters P s are in fact composition-independent within the statistical errors. The data points represent the average over >1,000 islands for each composition using STM images such as Fig. 4b that display apparent height contrast between Pt core and alloy shell. 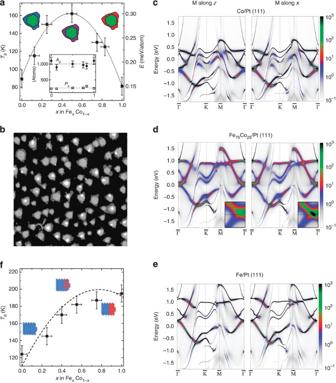Figure 4: Interline versus alloy anisotropy. (a)Tbmeasured for Pt core FexCo1−x-alloy shell islands. The dotted curve is a fit withE(x) described in the text. Sketches use colour code for the elements as in preceding figures. Inset: mean shell areaAsand perimeter lengthPsare independent ofx. (b) STM image (150 × 150 nm) of Pt core Fe0.5Co0.5-shell islands (Pt cores Θc=0.15 ML,FPt=0.007±0.001 ML min−1,Tdep=250 K,Tann=800 K; alloy shells: co-deposition of Θs=0.20 ML at 300 K). (c–e) Calculated band structures along the high symmetry directionof the surface Brillouin zone for the minority spin 3d-states of a pseudomorphic (c) Co, (d) Fe0.75Co0.25and (e) Fe monolayer on Pt(111). The colour code represents the intensity of the Bloch spectral function33in arbitrary units. (f)Tb(x) measured for Co core FexCo1−x-alloy shell islands. The dashed line shows a fit adding the experimentally determined Fe/Co interline contribution to the alloy anisotropy (Θc=0.12 ML, Θs=0.15 ML). Vertical error bars inaandfas inFig. 1, horizontal ones reflect the uncertainty of the flux calibration (Methods). Figure 4: Interline versus alloy anisotropy. ( a ) T b measured for Pt core Fe x Co 1− x -alloy shell islands. The dotted curve is a fit with E ( x ) described in the text. Sketches use colour code for the elements as in preceding figures. Inset: mean shell area A s and perimeter length P s are independent of x . ( b ) STM image (150 × 150 nm) of Pt core Fe 0.5 Co 0.5 -shell islands (Pt cores Θ c =0.15 ML, F Pt =0.007±0.001 ML min −1 , T dep =250 K, T ann =800 K; alloy shells: co-deposition of Θ s =0.20 ML at 300 K). ( c–e ) Calculated band structures along the high symmetry direction of the surface Brillouin zone for the minority spin 3 d -states of a pseudomorphic ( c ) Co, ( d ) Fe 0.75 Co 0.25 and ( e ) Fe monolayer on Pt(111). The colour code represents the intensity of the Bloch spectral function [33] in arbitrary units. ( f ) T b ( x ) measured for Co core Fe x Co 1− x -alloy shell islands. The dashed line shows a fit adding the experimentally determined Fe/Co interline contribution to the alloy anisotropy (Θ c =0.12 ML, Θ s =0.15 ML). Vertical error bars in a and f as in Fig. 1 , horizontal ones reflect the uncertainty of the flux calibration (Methods). Full size image The blocking temperature has the shape of an inverted parabola taking on its maximum at equi-atomic composition, where T b doubles with respect to the pure elements ( Fig. 4a ). This behaviour is very well described by the dotted curve displaying T b = E ( x )/ k B ln( v 0 / f ), with ν 0 and f as above, and with E ( x )= A s [ E Fe x + E Co (1− x )+ E a (1−4( x −0.5) 2 )]. This curve has three fit parameters. The first two are the shell averaged anisotropies of Co and Fe, determined by the left and right T b values to E Co =0.17±0.02 and E Fe =0.15±0.02 meV/atom, respectively. The third parameter is the additional energy barrier for thermal magnetization reversal created by the alloy and given by the maximum of the curve to E a =0.14±0.02 meV/atom. Our STM data reveal that also the alloy shells are pseudomorphic with the Pt(111) substrate for all compositions, that is they have constant strain. Their chemical order is very likely random because of the growth by co-deposition at room temperature, impeding thermal rearrangement of the atoms once they have attached to the islands. We address the origin of the anisotropy increase in the alloy by K mc calculations of Fe x Co 1− x islands. In line with previous calculations on Fe x Co 1− x monolayers [27] , we obtain the K mc maximum with x =0.75 at higher Fe content than in experiment. However, vertical relaxation yields with x =0.60, a value closer to experiment ( Supplementary Fig. S2 ). We find practically identical K mc ( x ) curves for alloy islands having as in experiment an interline to Pt, for pure alloy islands, and for an alloy monolayer ( Supplementary Fig. S3 ). Hence, the interline to Pt, as well as the atomic coordination number, do have a much smaller role in the alloy than in the clean elements and we can analyse the cause of the anisotropy for the monolayer, where the continuous band structure is accessible from the calculations. We find that spin–orbit coupling (SOC) lifts the degeneracy with respect to the magnetization direction of two bands deriving from in-plane orbitals with d xy and character ( Supplementary Fig. S4 ). When these spin-split states coincide with the Fermi level, the energy difference between both magnetization directions is maximum. As Fe has one d -electron less than Co, an increasing Fe content in the alloy generates a downward shift of E F , as clearly visible in Fig. 4c–e . At x =0.75 E F falls exactly in between the spin-split bands at the -point, whereas these bands lie fully below E F for pure Co and fully above for pure Fe. They are degenerate for in-plane magnetization, while for out-of-plane magnetization the d xy -derived band is pulled below and the states are pushed above E F , see the magnified view in the inserts in Fig. 4d . This results in a total energy minimum for out-of-plane magnetization. The anisotropy variation of the alloy is therefore a topological electronic effect, it is due to "hot spots" in the band structure. A very similar effect has been discussed for tetragonally distorted FeCo bulk alloys [34] . Similar, but much more pronounced effects of the electronic structure are also responsible for the large anisotropy changes in the core–shell islands, where the corresponding local density of states is highly sensitive to the chemistry of the neighbouring atomic species. Note that ‘hot spots’ resulting in very large K mc are also found for free-standing layers and for monolayers adsorbed onto the close-packed surfaces of other elements ( Supplementary Figs S4 and S5 and Supplementary Discussion). Figure 4f addresses to which extent alloy and interline effects can be added and shows T b ( x ) for five atom-wide Fe x Co 1− x shells placed around Co- instead of Pt cores. The Fe content changes the Co/Fe interline length and the alloy composition at the same time. For pure Co shells there is no interline between core and shell and T b is low, then it augments mainly due to the alloy anisotropy increasing with x . Further increase of the Fe concentration augments the Fe/Co interline length, making the islands magnetically harder, whereas the composition of the alloy goes beyond the ideal one. The superposition of both effects leads to a small increase for large x instead of the T b drop observed with Pt cores. The dashed line shows a quantitative analysis taking the Fe/Co interline value determined above plus an additional alloy anisotropy of E =0.11±0.02 meV/atom at x =0.50. This value and the ideal composition, compare well with the additional alloy anisotropy of E =0.14±0.02 meV per atom inferred for the Pt-core alloy–shell islands. This shows that the alloy anisotropy is independent of core chemistry and that alloy and interline anisotropy are additive. The fact that the experimental T b ( x ) values are monotonically increasing shows that a single atomically sharp Fe/Co interline has more anisotropy than a five atom-wide shell of a homogeneous FeCo alloy with ideal composition. 1D interlines versus 2D interfaces From Fig. 1 it has become evident that Co/Pt interfaces and interlines have very different anisotropies. We find that this directional and dimensional dependence of the interface anisotropy is particularly pronounced for the case of Co and Pd. 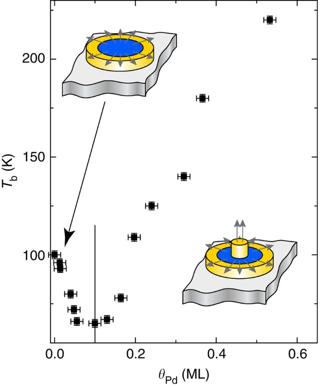Figure 5: Co/Pd interlines versus interfaces. The Pd atoms deposited onto the Pt terraces diffuse and laterally attach to the Co cores creating a Co/Pd interline decreasingTb. At ΘPd=0.1 ML this interline is completed, while the Pd islands forming on top of the Co cores creating a (111)-oriented Co/Pd interface continue to grow. This interface strongly increasesTb. Origin of error bars as inFig. 4. (Co core: Θc=0.07 ML atTdep=150 K, Θc=0.10 ML atTdep=250 K, Pd decoration:FPd=0.022±0.002 ML min−1,Tdep=250 K). Figure 5 shows T b (Θ Pd ) for Co-core islands that are decorated by Pd. One sees that T b has a minimum at 0.1 ML, from where on it steeply increases up to T b =220±5 K for Θ Pd =0.53 ML. This behaviour is attributed to the strongly differing saturation coverages for lateral versus vertical decoration. For the chosen deposition temperature, all the Pd atoms landing on the Pt terrace can diffuse to the Co islands. For homogeneous decoration they form a one atom-wide seam at 0.03 ML. At 0.1 ML this seam is on average three atoms wide and therefore the lateral decoration can be considered as being saturated for the magnetic interline properties. However, at this coverage, only 12% of the Co is decorated from the top, under the assumption of statistical growth and that all the Pd landing on Pd diffuses towards the Co core, as experimentally observed ( Supplementary Fig. S6 ). We therefore find that the Co/Pd interline reduces the anisotropy, similar to the edge decoration by Pt in Fig. 1 . From the minimum T b (0.10 ML)=65±5 K we derive E il, Co−Pd =−0.42±0.04 meV/atom, comparable to the value measured for Pt. For higher Pd coverage the Co core becomes progressively and selectively decorated by Pd from the top, see Supplementary Fig. S6 , and we derive an interface-induced increase of E if, Co−Pd =0.38±0.04 meV/atom. This is in good agreement with the value of E if, Co−Pd =0.4 meV/atom calculated for a monolayer sequence of Pd/Co/Pd(111) [17] and experimentally derived from the thickness-dependent anisotropy of Co films in Pd/Co/Pd(111) sandwiches [16] , [35] , [36] . The present results reveal that a single Pd monolayer suffices for the Co/Pd interface anisotropy to fully develop. Again, because Pd and Pt have almost identical lattice constant, we expect strain effects to be small. Supplementary Figs S6 and S7 show that morphological and magnetic island coalescence can be excluded. Figure 5: Co/Pd interlines versus interfaces. The Pd atoms deposited onto the Pt terraces diffuse and laterally attach to the Co cores creating a Co/Pd interline decreasing T b . At Θ Pd =0.1 ML this interline is completed, while the Pd islands forming on top of the Co cores creating a (111)-oriented Co/Pd interface continue to grow. This interface strongly increases T b . Origin of error bars as in Fig. 4 . (Co core: Θ c =0.07 ML at T dep =150 K, Θ c =0.10 ML at T dep =250 K, Pd decoration: F Pd =0.022±0.002 ML min −1 , T dep =250 K). 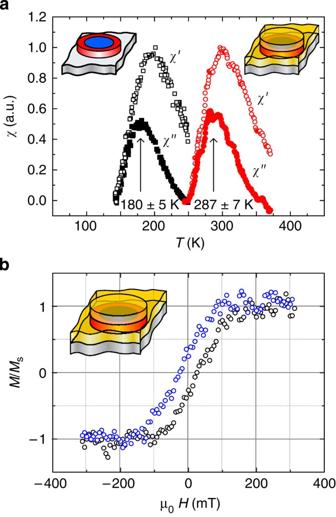Figure 6: Combination of interline and interface effects approaching room temperature blocking. (a) Real (χ′(T)) and imaginary part (χ″(T)) of the zero-field magnetic susceptibility shown as empty and filled symbols, respectively.. Black: Co-core Fe-shell islands, red: after capping with 1 ML Pd. The curves have been normalized such that the maximum of χ′(T) is unity, the actual signal decreases by a factor of 1.6 by capping. (b) Magnetization curve for increasing (black) and decreasing field (blue) of the CoFePd islands showing hysteresis atT=250 K. (ΘCo=0.07 ML,Tdep=150 K, ΘCo=0.10 ML,Tdep=250 K; ΘFe=0.09 ML,Tdep=250 K; ΘPd=1.0 ML,Tdep=100 K,Tann=250 K). Full size image We demonstrate in Figure 6 that the interline anisotropy survives upon capping, and thus the orientation and chemistry-dependent interline and interface magnetic anisotropies can be added up for three elements in contact with Co, such as to maximize T b for a given size. Fig. 6a shows the real and imaginary parts of the out-of-plane susceptibility of Co-core islands surrounded by Fe shells without (black) and with (red) a Pd cap monolayer. The Pd capping, when performed at low deposition temperature with subsequent annealing, essentially replicates the morphology of the initial surface before capping. T b is seen to increase by Pd capping from 180±5 to 287±7 K. Thus, combining interline and interface anisotropy brings one from 100 K for a pure Co island to almost 300 K for an island with an Fe/Co interline and a Co/Pd top interface. The out-of-plane M ( H )-curve shown in Fig. 6b displays magnetic remanence at 250 K. Owing to the longer time scale of the M ( H ) measurement compared with the one of χ( T ), one has to go to lower T than T b to observe remanence. Supplementary Fig. S8 shows that Pd capping does not induce magnetic coalescence. Figure 6: Combination of interline and interface effects approaching room temperature blocking. ( a ) Real (χ′( T )) and imaginary part (χ″( T )) of the zero-field magnetic susceptibility shown as empty and filled symbols, respectively.. Black: Co-core Fe-shell islands, red: after capping with 1 ML Pd. The curves have been normalized such that the maximum of χ′( T ) is unity, the actual signal decreases by a factor of 1.6 by capping. ( b ) Magnetization curve for increasing (black) and decreasing field (blue) of the CoFePd islands showing hysteresis at T =250 K. (Θ Co =0.07 ML, T dep =150 K, Θ Co =0.10 ML, T dep =250 K; Θ Fe =0.09 ML, T dep =250 K; Θ Pd =1.0 ML, T dep =100 K, T ann =250 K). Full size image Our results are a significant step towards atomic-scale materials science and engineering of magnetic nanostructures using the magnetic hardness emerging from 2D interfaces between single atomic layers and 1D interlines involving only a few atom-wide shells. Most of the element combinations employed in the present study follow the classical rule, where magnetic 3 d elements, such as Co and Fe, are combined with 4 d and 5 d elements with high SOC and magnetic polarizability, such as Pd and Pt (refs 15 , 37 , 38 ). However, we find a number of surprises. Interfacing two elements with low SOC, namely Fe and Co, leads to high out-of-plane interline anisotropy such that onion-type alternations of the two elements with shell thicknesses of five atoms or less are giving higher hardness than a homogeneous alloy. For all elements we find an unexpected strong dependence of the interface anisotropy on crystallographic orientation and dimension. Co/Pt and Co/Pd 2D interfaces with {111}-orientation induce strong anisotropy along 111 , whereas 1D interlines between the same elements with their normal oriented in the 111 plane strongly reduce this anisotropy. Tentatively, one can explain this behaviour by the Co/Pt and Co/Pd interlines wanting the magnetization to point perpendicular to them, as schematically indicated by the arrows in Figs 1 and 5 . The circular average over the interline around the core gives a vanishing in-plane, but a reduced out-of-plane anisotropy. Co/Fe interlines have opposite directional dependence of the induced anisotropy, that is, they want the magnetization to point perpendicular to the interline and along 111 , giving the observed increase of the out-of-plane anisotropy. This difference between interlines and interfaces emphasizes the importance of the directional hybridization for the resulting anisotropy and straightforwardly explains that an arrangement of alternating atomic Fe and Pt rows [39] exhibits quite different magnetic properties than the alternating close-packed planes of these elements in the highly anisotropic L1 0 phase. Our calculations show that the effects are of electronic origin and that one needs to consider the spin- and k- -resolved electronic structure in detail to determine in which crystallographic directions the hot spots at E F are located. This can be very sensitive to little changes of the lattice constant, explaining why only specific lattice distortions give rise to the desired high anisotropies in CoFe [34] , [40] or CoPt and FePt [41] , [42] alloys. The interline anisotropies reported here are by an order of magnitude larger than the ones reported for Co double-layer islands decorated by Au [21] . The variation of the magnetic anisotropy reported for Pt decoration of Co double-layer islands on Au(111) with increasing Pt coverage is qualitatively similar to the variation of T b we see for Pd decoration; however, the amplitudes are again significantly smaller [43] . The potential of the present results in the atomic-scale design of future magnetic recording materials [44] , [45] can be assessed by comparing our numbers with the highest hardnesses achieved in FePt colloidal nanoparticles or grains in sputter-deposited FePt media. In both cases, the particles can only partly be transformed to the L1 0 phase without coalescence, giving rise to an effective magnetic anisotropy significantly below the L1 0 bulk value. For colloidal particles the highest reported value is K eff =0.30 meV/unit cell [42] and for granular media K eff =0.45 meV per unit cell [46] . These numbers are smaller or comparable to the ones reported in this paper for the interline and interface anisotropies. Evidently, the present structures are 2D and thus laterally larger than the 3D particles and our results have to be transferred to 3D to create the ultimate bit sizes. The good agreement of the general trends between experiment and state-of-the-art theory opens the door for a fundamental understanding of interface and interline-induced magnetic anisotropy and encourages ab-initio -aided design of magnetic nanostructures. Synthesis and Characterization The bi- and tri-metallic nanostructures have been grown by atomic beam epitaxy under ultra-high vacuum (UHV) in a chamber with a base pressure of p tot ≤3 × 10 −11 mbar and a pressure during growth of p tot ≤8 × 10 −11 mbar. The chamber has been designed to perform growth, MOKE and STM measurements with the sample held at the same position enabling full control of its temperature (40–1,400 K) throughout any of the growth and characterization steps [30] , [47] . This has been essential as the growth morphologies have been achieved by kinetic control [32] , that is, by the careful choice of deposition and annealing temperatures for each element, and depending on whether it is used for growing the core, shell or cap layer. These temperatures, as well as the used coverages and deposition fluxes, are given for each case in the figure captions. Atomically sharp vertical interfaces have been ensured by staying below the temperatures, where insertion into or exchange with the Pt(111) substrate sets in. This temperature is lower for the adatoms present during growth than for an adsorbed island or a thin film. As an example, the values for Co/Pt(111) are T ins, atom =180 K (ref. 48 ) and T ex, monolayer =375 K (ref. 49 ), respectively. Atomically sharp lateral interlines have been ensured by keeping the annealing and deposition temperatures below the ones where lateral inter-diffusion sets in. STM images with chemical contrast enable to control the absence of vertical and lateral inter-diffusion. However, also the magnetic properties are very sensitive indicators for such site-exchange processes. They show up by irreversible χ( T ) curves, sometimes the magnetic hardness is even increased by passing the reversible temperature, but as the morphology is then no more controlled on the atomic scale we chose the upper temperature of the χ( T ) measurements such that they are fully reversible, therefore preserving atomically sharp interfaces. The island cores have been created by nucleation at the temperature giving the desired island density for the applied flux, adatom diffusion barriers and attempt frequencies specific to each element [32] . Owing to limited-edge diffusion the islands have fractal shape and subsequent annealing makes them more compact. For the Pt cores we annealed to high temperature to achieve the 2D thermodynamic equilibrium island shape bound by straight atomic steps running along the crystallographic directions. Opposite steps are non-equivalent and their respective length is given by their step-free energies leading to quasi-hexagons. For the Co cores the annealing temperature is limited to T ann =250 K by the fact that double-layer islands form from 320 K on and Co diffusion into Pt sets in at 375 K (ref. 49 ). Consequently, the Co cores do not have the thermodynamic equilibrium shape. The shell growth requires a sufficiently large adatom diffusion path such that all atoms deposited between the cores can join them; it further requires interlayer diffusion of atoms landing on the cores down to the substrate, and finally thermally activated insertion into the substrate has to be avoided. Therefore, the deposition temperature for the shell elements is given by the compromise between the first two and the last requirements. We limited the total coverage of cores and shells for the compact Pt cores to 0.35 ML and for the more elongated Co cores to 0.30 ML to have negligible coalescence [32] . For the alloy shell the Fe and Co fluxes were adjusted to yield the desired stoichiometry for co-deposition of both elements. For each element, the flux calibration was done by evaporating on the clean Pt(111) surface an amount of material roughly equivalent to Θ=0.4 ML. The exact covered area has then been estimated by STM. The uncertainty of this number is given by tip-convolution effects, which are low for compact growth morphologies and therefore deposition has been taken out at room temperature. The uncertainty in the open-shutter time contributes less to the error as the evaporation times have been with >1 min relatively long. Owing to the large number of low-coordinated atoms, being highly reactive but at the same time deterministic for the magnetic properties [30] , the samples are very sensitive to the residual gas and we detect a change of the magnetic properties in the most sensitive cases already 1 h after deposition, despite the low base pressure. Therefore, the MOKE measurements have been performed directly after growth. For the same reasons a fresh sample had been prepared for each of the T b measurements. The MOKE measurements of χ( T ) have been performed in polar geometry with an out-of-plane field of H = H 0 sin(2π ft ) with H 0 =100 Oe, f =11 Hz, and lock-in detection to measure the real and imaginary parts of the zero-field susceptibility, χ′( T ) and χ″( T ), respectively. Taking into account the island size distribution, the islands that give the highest susceptibility signal are the ones with 1.65 times the average size. The acquisition time for the magnetization loops shown in Fig. 6b has been 300 s. Theoretical Calculations For the spin-polarized, fully relativistic calculations we have employed our implementation of the Korringa–Kohn–Rostoker Green’s function method where the electron density is calculated self-consistently within the local spin density approximation using spherical potentials. Because the formalism is based on the four-component Dirac equation it gives direct access to spin–orbit-induced properties such as orbital magnetic moments and the magneto-crystalline anisotropy energy K mc . Owing to the higher numerical accuracy we performed magnetic torque calculations to derive K mc [50] , [51] . How to cite this article: Ouazi, S. et al . Atomic scale engineering of magnetic anisotropy of nanostructures through interfaces and interlines. Nat. Commun . 3:1313 doi: 10.1038/ncomms2316 (2012).